Stereoselective synthesis of medium lactams enabled by metal-free hydroalkoxylation/stereospecific [1,3]-rearrangement Rearrangement reactions have attracted considerable interest over the past decades due to their high bond-forming efficiency and atom economy in the construction of complex organic architectures. In contrast to the well-established [3,3]-rearrangement, [1,3] O-to-C rearrangement has been far less vigorously investigated, and stereospecific [1,3]-rearrangement is extremely rare. Here, we report a metal-free intramolecular hydroalkoxylation/[1,3]-rearrangement, leading to the practical and atom-economical assembly of various valuable medium-sized lactams with wide substrate scope and excellent diastereoselectivity. Moreover, such an asymmetric cascade cyclization has also been realized by chiral Brønsted acid-catalyzed kinetic resolution. In addition, biological tests reveal that some of these medium-sized lactams displayed their bioactivity as antitumor agents against melanoma cells, esophageal cancer cells and breast cancer cells. A mechanistic rationale for the reaction is further supported by control experiments and theoretical calculations. Eight-membered lactams, especially the benzo[ d ]azocinones, are prominent structural motifs that can be found in many natural products and bioactive molecules (Fig. 1 ) [1] , [2] , [3] , [4] , [5] . However, access to these heterocycles is challenging owing to unfavorable enthalpic and entropic barriers in transition states leading to medium-sized rings [6] , [7] , [8] , [9] , [10] . To date, only very limited methods have been developed, and most of them rely on noble-metal catalysis [11] , [12] , [13] , [14] , [15] , [16] , [17] , [18] , [19] . To this end, the development of new methods for the efficient construction of this skeleton is highly desirable, especially those with high diastereo- and enantioselectivity. Fig. 1 Benzo[ d ]azocinones in natural products and bioactive molecules. Some of representative molecules are listed Full size image Rearrangement reactions have attracted considerable interest over the past decades due to their high bond-forming efficiency and atom economy in the construction of complex organic architectures [20] , [21] . In contrast to the well-established [3,3]-rearrangement [22] , [23] , [24] , [25] , which generally proceeds via the chair-like transition state and thus is stereospecific (Figs. 2a ), [1,3] O-to-C rearrangement has been far less vigorously investigated, and stereospecific [1,3]-rearrangement is highly challenging due to the formation of presumable zwitterion pairs (Fig. 2b ) [26] , [27] . Although several Lewis acid-mediated and thermal [1,3]-rearrangements that relay stereochemical information have been reported [28] , [29] , transformation in these limited cases lacks generality and significant deterioration of enantiomeric excess is observed [30] , [31] . Fig. 2 [3,3]-Rearrangement vs. [1,3]-rearrangement. a Typical [3,3]-rearrangement. b Typical [1,3]-rearrangement. c This work: Brønsted acid-catalyzed hydroalkoxylation/stereospecific [1,3]-rearrangement Full size image Recently, great progress of transition metal-catalyzed intramolecular alkoxylation-initiated [1,3]-rearrangement has evoked a new round of exploration on the [1,3]-rearrangements, offering great potential to build structurally complex cyclic molecules, as elegantly established by Toste, Rhee, Hashmi, Liu, Davies, and Zhu [31] , [32] , [33] , [34] , [35] , [36] , [37] , [38] . Despite these impressive advances, these tandem reactions are limited to ether nucleophiles and rely on noble metals (Au/Pt) as the catalyst. Importantly, no direct catalytic asymmetric tandem reaction has been described to date [39] . Inspired by the above results and by our recent study on yttrium-catalyzed tandem intramolecular hydroalkoxylation/Claisen rearrangement [40] , we envisioned that the synthesis of eight-membered benzo[ d ]azocinones 2 might be accessed directly through catalytic intramolecular hydroalkoxylation/[1,3]-rearrangement of ynamides 1 [41] , [42] , [43] , [44] , [45] , [46] , [47] , [48] , [49] , [50] . Herein, we describe the realization of a metal-free tandem intramolecular hydroalkoxylation/[1,3]-rearrangement (Fig. 2c ), and this method leads to the practical and atom-economical synthesis of various valuable medium-sized lactams with excellent diastereoselectivity. Moreover, such an asymmetric cascade cyclization has also been achieved via kinetic resolution by chiral spiro phosphoramide catalysis. Importantly, this [1,3]-rearrangement is highly stereospecific and proceeds with complete chirality transfer. Control experiments and density functional theory (DFT) calculations provide further evidence of the feasibility of the proposed mechanism. 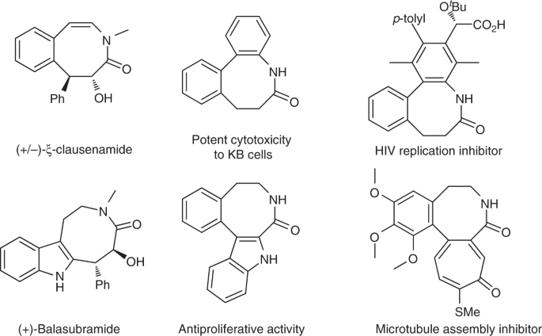Fig. 1 Benzo[d]azocinones in natural products and bioactive molecules. Some of representative molecules are listed Screening of reaction conditions At the outset, ynamide 1a was used as the model substrate to demonstrate our designed cascade cyclization, as shown in Table 1 (for more details see Supplementary Table 1 ). To our delight, the expected benzo[ d ]azocinone 2a was indeed formed with exclusive cis -diastereoselectivity (diastereoselectivity (d.r.) >50:1; determined by crude proton nuclear magnetic resonance ( 1 H NMR)), albeit in low yields, in the presence of typical gold catalysts (Table 1 , entries 1 and 2). Somewhat surprisingly, further investigations revealed that the reaction also proceeded in the presence of various non-noble metals (Table 1 , entries 4–7), with Zn(OTf) 2 giving the best yield of the desired product 2a (Table 1 , entry 7). In addition, Brønsted acids such as TsOH and MsOH could also catalyze this cascade reaction to produce 2a in 47 and 66% yields, respectively, together with significant amounts of hydration product 2a′ in both cases (Table 1 , entries 8 and 9). Although the use of 10 mol% of HOTf as catalyst failed to produce the desired 2a , probably because the high acidity led to decomposition of 1a (Table 1 , entry 10), the reaction efficiency was substantially improved by decreasing the loading of catalyst (Table 1 , entries 11–13). With a low catalyst loading of 0.5 mol%, HOTf efficiently catalyzed the formation of 2a in 96% yield (Table 1 , entry 13). These results indicate that HOTf, which was released as a hidden Brønsted acid, is presumably the true catalytic species in the above Lewis acid catalysis [51] , [52] , [53] . Table 1 Optimization of reaction conditions a Full size table Reaction scope study The reaction scope was then explored under the optimized reaction conditions (Fig. 3 ). This metal-free tandem reaction occurred efficiently with various benzyl alcohol-tethered ynamides 1 , leading to the corresponding benzo[ d ]azocinones 2 in good to excellent yields. Importantly, excellent diastereoselectivity (>50:1) was achieved in all cases. Ynamides with different sulfonyl-protecting groups were first investigated, and the desired products 2a – 2c were formed in 73–94% yields. In addition, ynamides bearing either electron-withdrawing or electron-donating substituents, such as F, Cl, Br, Me, OMe, or even CN and CF 3 on the aromatic ring (R 2 = Ar), were compatible with this cyclization to produce the expected 2d – 2l in generally excellent yields. This cascade cyclization was also extended to the naphthalene, thiophene, and alkenyl-substituted ynamides, delivering the desired 2m (99%), 2n (81%), and 2o (94%), respectively. Various aryl-substituted ynamides with either electron-donating or electron-withdrawing groups were then screened, and the reaction afforded the desired products 2p – 2ab in 73–98% yields. Of note, in some cases better yields could be achieved by employing Zn(OTf) 2 (10 mol%) as catalyst and 5 Å molecular sieve (MS) as additive ( 2s and 2aa ). Interestingly, alkyl-substituted ynamides (R 1 or R 2 = alkyl) were also suitable substrates, and were converted into the desired 2ac and 2ad in good yields, and 2ae in a serviceable yield; higher temperature was needed in these cases. The molecular structures of 2a and 2ac were confirmed by X-ray diffraction (for more details see Supplementary Tables 3 and 4 ). Fig. 3 Reaction scope for the formation of 3-benzazocinones 2 . Reaction conditions: 1 (0.2 mmol), HOTf (0.001 mmol), PhCl (4 mL), 80 °C, 4 h, in vials; yields are those for the isolated products. a 1 mol% of HOTf was used. b Using 10 mol% of Zn(OTf) 2 as catalyst and 5 Å molecular sieve (MS) as additive. c 100 °C, 60 h. d 100 °C, 4 h Full size image Notably, this cascade cyclization was also extended to the allyl alcohol-tethered ynamides, and, importantly, no competing intramolecular hydroalkoxylation/[3,3]-rearrangement was observed [40] . As shown in Fig. 4a , the desired benzo[ d ]azocinones 2af – 2ah were obtained in 61–76% yields, and significantly improved yield (86%) was achieved in case of ynamide 1ah by using Zn(OTf) 2 as catalyst. In addition, the reaction proceeded smoothly to produce the expected 9-membered lactam 2ai in 46% yield, and, in this case, the use of Zn(OTf) 2 as catalyst also gave significantly improved yield (Fig. 4b , 2ai was confirmed by X-ray diffraction, for more details see Supplementary Table 5 ). Moreover, it was found that other heterocycle-linked 8-membered ring lactams 2aj – 2am could also be synthesized in 41−55% yields in the presence of 20 mol% of HNTf 2 as catalyst (Fig. 4c ). 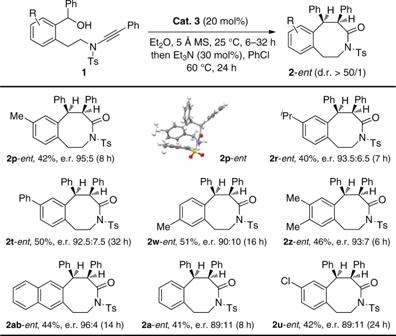Fig. 5 Reaction scope for kinetic resolution of racemic1. Reaction conditions:1(0.1 mmol),Cat.3(0.02 mmol), Et2O (2 mL), 25 °C, 6–32 h, then Et3N (0.03 mmol), PhCl (1 mL), 60 °C, 24 h, in vials; yields are those for the isolated products; e.r.s are determined by high-performance liquid chromatography (HPLC) analysis on a chiral stationary phase Attempts to extend the reaction to the terminal ynamide 1an only gave a complex mixture of products, and the reaction of ynamides 1ao and 1ap also failed to produce the desired products (for more details see Supplementary Figs. 118 and 119 ), indicating that the formation of a stable benzylic carbocation is a key requirement for subsequent [1,3]-rearrangement (Fig. 4d ). Fig. 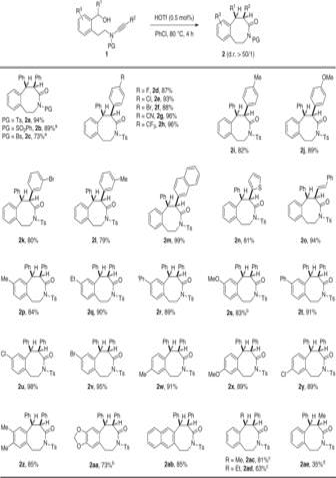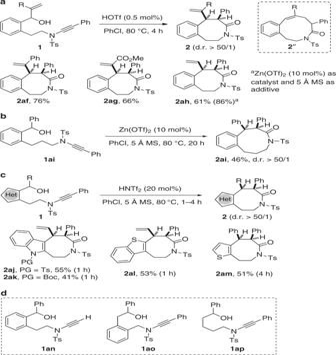4 Catalytic hydroalkoxylation/[1,3]-rearrangement of other ynamides 1 . Fig. 4 Catalytic hydroalkoxylation/[1,3]-rearrangement of other ynamides1.aBrønsted acid-catalyzed hydroalkoxylation/[1,3]-rearrangement of allyl alcohol-tethered ynamides1af–1ah.bZinc-catalyzed cascade cyclization of ynamide1ai.cHNTf2-catalyzed cascade cyclization of other heterocycle-linked ynamides1aj–1am.dYnamides1an–1apwhich failed to give the desired products Fig. 3 Reaction scope for the formation of 3-benzazocinones2. Reaction conditions:1(0.2 mmol), HOTf (0.001 mmol), PhCl (4 mL), 80 °C, 4 h, in vials; yields are those for the isolated products.a1 mol% of HOTf was used.bUsing 10 mol% of Zn(OTf)2as catalyst and 5 Å molecular sieve (MS) as additive.c100 °C, 60 h.d100 °C, 4 h a Brønsted acid-catalyzed hydroalkoxylation/[1,3]-rearrangement of allyl alcohol-tethered ynamides 1af – 1ah . 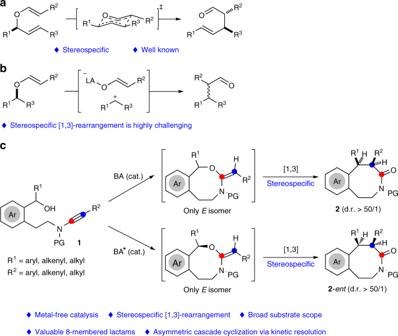b Zinc-catalyzed cascade cyclization of ynamide 1ai . c HNTf 2 -catalyzed cascade cyclization of other heterocycle-linked ynamides 1aj – 1am . d Ynamides 1an – 1ap which failed to give the desired products Full size image Screening of reaction conditions for kinetic resolution We then considered the possibility of developing an asymmetric variant of this tandem sequence. Fig. 2 [3,3]-Rearrangement vs. [1,3]-rearrangement.aTypical [3,3]-rearrangement.bTypical [1,3]-rearrangement.cThis work: Brønsted acid-catalyzed hydroalkoxylation/stereospecific [1,3]-rearrangement Although no enantioselectivity was observed by the use of chiral metal catalysts, good enantioselectivity could be attained by employing chiral spiro phosphoramides as catalysts (for more details, see Supplementary Table 2 and Supplementary Fig. 120 ) [54] , [55] . Importantly, further studies revealed that the chiral induction was realized through kinetic resolution of racemic ynamides (for more details, see Supplementary Fig. 121 ). Initially, ynamide 1p , bearing an electron-donating methyl group on the aromatic ring moiety that should promote this cascade cyclization, was used as the model substrate. As shown in Table 2 , the desired chiral benzo[ d ]azocinone 2p - ent was obtained in 42% yield with an enantiomeric ratio (e.r.) of 95:5 in the presence of chiral spiro phosphoramide Cat. 3 [56] , [57] , [58] , [59] , bearing two 6,6'-di(3,5-di- tert -butyl-4-methoxyphenyl) moieties (Table 2 , entry 5). Interestingly, the use of the corresponding chiral binol-derived phosphoramide led to significantly decreased enantioselectivity (e.r. <60:40), indicating that the spirobiindane backbone of the phosphoramides plays a crucial role in the chiral induction step. It is notable that in this process one enantiomer (( R )- 1p ) favored formation of the desired chiral benzo[ d ]azocinone 2p - ent , while the other enantiomer (( S )- 1p ), which does not match with the Cat. 3 , favored formation of the corresponding hydration product 2p' catalyzed by the acid (for more details, see Supplementary Figs. 122 – 124 ). Thus, it represents a rare example of parallel kinetic resolution [60] , [61] . Table 2 Kinetic resolution of racemic 1p with chiral spiro phosphoramides a Full size table Scope of kinetic resolution of racemic ynamides 1 Preliminary investigations were carried out into the reaction scope by employing chiral spiro phosphoramide Cat. 3 as a catalyst (Fig. 5 ). Substrates with either electron-donating or electron-withdrawing groups on the aromatic ring moiety of the racemic ynamides 1 were well tolerated and resulted in 40–51% yields and good e.r. values. 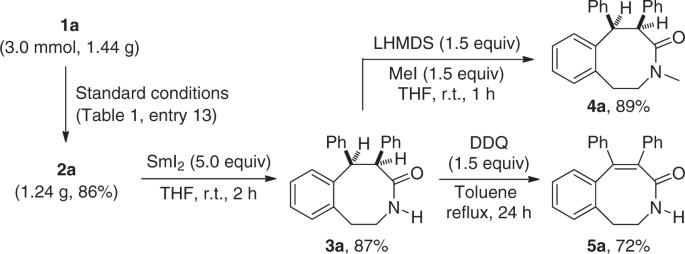Fig. 6 Gram-scale reaction and product elaboration. Gram-scale reaction of ynamide1aand transformation of2ainto3a,4a, and5a The absolute configuration of 2p - ent was determined by X-ray crystallographic analysis (for more details, see Supplementary Table 6 ). Of note, although 20 mol% catalyst loading was employed, probably because the acidity of the chiral catalyst is not high enough, the catalyst could be readily recovered and reused five times with almost unchanged enantioselectivity and reactivity (for more details, see Supplementary Fig. 125 ). 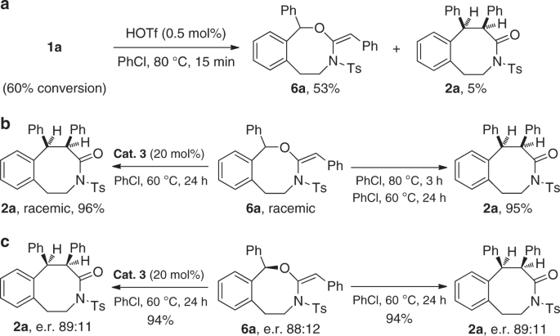Fig. 7 Control experiments.aCascade cyclization of ynamide1aby quenching the reaction after 15 min.bControl experiments on the transformation of racemic6ainto racemic2a.cControl experiments on the transformation of chiral6ainto chiral2a Fig. 5 Reaction scope for kinetic resolution of racemic 1 . Reaction conditions: 1 (0.1 mmol), Cat. 3 (0.02 mmol), Et 2 O (2 mL), 25 °C, 6–32 h, then Et 3 N (0.03 mmol), PhCl (1 mL), 60 °C, 24 h, in vials; yields are those for the isolated products; e.r.s are determined by high-performance liquid chromatography (HPLC) analysis on a chiral stationary phase Full size image Synthetic applications and biological tests To further demonstrate the potential utility of this reaction, we also carried out product derivatizations (Fig. 6 ). For example, the Ts group in benzo[ d ]azocinone 2a , prepared on a gram scale in 86% yield, was efficiently removed to form free amide 3a in 87% yield by the treatment with SmI 2 . 3a could be further methylated into the corresponding lactam 4a (89%) and oxidized into unsaturated lactam 5a (72%), respectively. Fig. 6 Gram-scale reaction and product elaboration. Gram-scale reaction of ynamide 1a and transformation of 2a into 3a , 4a , and 5a Full size image Moreover, we tested the above-synthesized 3-benzazocinones for their bioactivity as antitumor agents. The cytotoxic effects of these compounds were evaluated against a panel of cancer cells, including melanoma cells A375, esophageal cancer cells SK-GT-4 and KYSE-450, and breast cancer cells MCF-7 and MDA-MB-231 using cell viability assay. 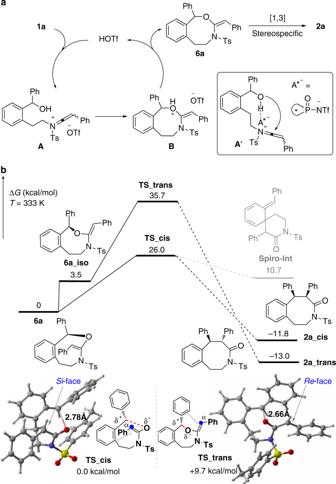Fig. 8 Mechanistic hypothesis.aPlausible catalytic cycle.bDensity functional theory (DFT) calculations on the O-to-C rearrangement of (R)-6a Our preliminary studies showed that almost half of these compounds exerted significant cytotoxic effects on the A375, and a few compounds ( 2ac , 2ah , 2p - ent , and 3a ) and compound 2am exerted cytotoxic effects on the SK-GT-4 and MCF-7 (for more details, see Supplementary Table 8 ), respectively, suggesting a potential application of these medium-sized lactams in medicinal chemistry. Mechanistic investigations We then turned our attention to mechanistic investigations (for more details, see Supplementary Figs. 126 – 129 ). First, it was found that no incorporation of 18 O into the product 2a was observed when ynamide 1a was subjected to the reaction conditions with H 2 18 O, which indicates that the oxygen on the carbonyl group of 2a originates from the hydroxyl group of 1a (for more details, see Supplementary Fig. 126 ). In addition, hydration product 2a′ was not converted into 2a under the standard conditions, thus ruling out 2a′ as a possible intermediate (for more details, see Supplementary Fig. 127 ). Gratifyingly, the ketene aminal 6a (only the E isomer) could be isolated in 53% yield by quenching the reaction after 15 min (Fig. 7a ). Importantly, 6a was readily converted into the desired 2a and complete chirality transfer was observed starting from chiral 6a (Fig. 7b, c ). Furthermore, the acid catalyst did not work in this rearrangement process, indicating that it is an uncatalyzed thermal rearrangement (for more details, see Supplementary Fig. 128 ). These results strongly support that 6a is the key intermediate and stereospecific [1,3]-rearrangement is presumably involved in this tandem process. Fig. 7 Control experiments. a Cascade cyclization of ynamide 1a by quenching the reaction after 15 min. b Control experiments on the transformation of racemic 6a into racemic 2a . c Control experiments on the transformation of chiral 6a into chiral 2a Full size image On the basis of the above observations, we propose a mechanism for the formation of benzo[ d ]azocinone 2a (Fig. 8 ). The reaction begins with the hydroxyl group attack of the HOTf-activated ynamide 1a to afford oxonium intermediate B presumably via a keteniminium intermediate A , thus further yielding thermodynamically stable vinyl ether intermediate 6a of E configuration and regenerating the acid catalyst. DFT calculations at B3LYP-D3/6-31G(d,p)//SMD-def2-TZVP level of theory [62] , [63] , [64] , [65] (for more details, see Supplementary Figs. 111 – 113 and Supplementary Datasets 1 – 4 ) were introduced to understand the subsequent O-to-C rearrangement of ( R )- 6a , which is a stereospecific, rate-determining, and uncatalyzed thermal rearrangement, to produce the final cis product ( R , S )- 2a . Two major conformational isomers of initial compound 6a and 6a-iso can be located by calculations in terms of different Si - or Re -face at the α-carbon of amide substrate. In the following step of C-O bond cleavage, transition state TS_cis with bond breaking via Si -face side was 9.7 kcal/mol more stable than that via Re -face cleavage-formed TS_trans , suggesting the final 2a_cis from TS_cis is kinetically favorable and highly stereospecific. Furthermore, calculations indicate that the reaction mechanism is not a typical [1,3]-rearrangement (for more details, see Supplementary Figs. 114 – 117 ) [66] , [67] , [68] , [69] , [70] . We are able to locate the transition states of C-O bond cleavage, but failed to locate transition states of C-C bond formation, which indicate that the mechanism seems not to be stepwise. Quantitative Sensory Testing method was used and three levels of methods (B3LYP-D3, M062X, ωB97XD) were tried in our calculations. All of them give substantially similar kinetic and thermodynamic results (for more details, see Supplementary Figs. 111 – 117 ). However, more inspections for transition states imply that the developing negative charge on the α-carbon of amide substrate tends to be stabilized by aromatic rings forming formal [3,3]-rearrangement transition states. A regular spiro[5,5] product spiro-int is not accessible because of its high energy instability for 22.5 kcal/mol, compared to the energy of 2a-cis . Indeed, transition states of C-C bond formation are facile to the final product during our calculations. Based on energy profiles, the pathway to form favorable 2a-cis is kinetically irreversible and thermodynamically exothermic for 11.8 kcal/mol, which is in agreement with our experiment. When chiral Brønsted acid is employed, the resulting keteniminium intermediate A′ leads to chiral 6a via ion pairing and H-bonding interactions [54] , [55] , which undergoes stereospecific [1,3]-rearrangement to form 2a - ent with complete chirality transfer. Fig. 8 Mechanistic hypothesis. a Plausible catalytic cycle. b Density functional theory (DFT) calculations on the O-to-C rearrangement of ( R )- 6a Full size image In summary, we have achieved a metal-free intramolecular hydroalkoxylation/[1,3]-rearrangement, and significantly, this [1,3]-rearrangement is highly stereospecific, and a mechanistic rationale for this stereospecificity is also strongly supported by DFT calculation. This method leads to the practical and atom-economical synthesis of a diverse array of valuable medium-sized lactams from readily available ynamides in high yields with broad substrate scope and excellent diastereoselectivity. Furthermore, this asymmetric cascade cyclization has also been realized via kinetic resolution by chiral spiro phosphoramide catalysis, thus constituting a rare example of chiral Brønsted acid-catalyzed kinetic resolution. In addition, biological tests reveal that some of these medium-sized lactams displayed their bioactivity as antitumor agents against melanoma cells, esophageal cancer cells, and breast cancer cells. We anticipate that the mechanistic insights of this chemistry may provoke new developments in related stereospecific [1,3]-rearrangement and chiral Brønsted acid-catalyzed kinetic resolution, and the present protocol will find broad applications in synthetic and medicinal chemistry. Materials Unless otherwise noted, materials were obtained commercially and used without further purification. All the solvents were treated according to general methods. Flash column chromatography was performed over silica gel (300–400 mesh). See Supplementary Methods for experimental details. General methods 1 H NMR spectra and carbon-13 nuclear magnetic resonance ( 13 C NMR) spectra were recorded on a Bruker AV-400 spectrometer and a Bruker AV-500 spectrometer in chloroform- d 3 . For 1 H NMR spectra, chemical shifts are reported in p.p.m. with the internal tetramethylsilane signal at 0.0 p.p.m. as a standard. For 13 C NMR spectra, chemical shifts are reported in p.p.m. with the internal chloroform signal at 77.0 p.p.m. as a standard. Infrared spectra were recorded on a Nicolet AVATER FTIR330 spectrometer as thin film and are reported in reciprocal centimeter (cm −1 ). Mass spectra were recorded with Micromass QTOF2 Quadrupole/Time-of-Flight Tandem mass spectrometer using electron spray ionization. 1 H NMR, 13 C NMR, and HPLC spectra (for chiral compounds) are supplied for all compounds: see Supplementary Figs. 1 – 110 . See Supplementary Methods for the characterization data of compounds not listed in this part. General procedure for the synthesis of 3-benzazocinones 2 To a mixture of the ynamide 1 (0.20 mmol) in PhCl (3.75 mL) at room temperature, HOTf (0.001 mmol/0.25 mL) in 0.25 mL PhCl was added. Then, the reaction mixture was stirred at 80 °C and the progress of the reaction was monitored by thin layer chromatography (TLC). The reaction typically took 4 h. Upon completion, the mixture was concentrated and the residue was purified by chromatography on silica gel (eluent: hexanes/ethyl acetate) to afford the desired 3-benzazocinone 2 . General procedure for the synthesis of chiral 2- ent To a mixture of the ynamide 1 (0.1 mmol) and 5 Å MS (60 mg) in Et 2 O (2 mL) at room temperature, Cat. 3 (0.02 mmol, 17.6 mg) was added during stiring. Then, the reaction mixture was stirred at 25 °C and the progress of the reaction was monitored by TLC. After the corresponding reaction time (6–32 h), Et 3 N (0.03 mmol, 4.2 μL) and PhCl (1 mL) was added to the reaction mixure to quench the Cat. 3 . The resulting reaction solution was stirred at 60 °C for another 24 h. The mixture was concentrated and the residue was purified by chromatography on silica gel (eluent: hexanes/ethyl acetate) to afford the desired chiral 3-benzazocinone 2 - ent .